Engineering chiral porous metal-organic frameworks for enantioselective adsorption and separation The separation of racemic molecules is of substantial significance not only for basic science but also for technical applications, such as fine chemicals and drug development. Here we report two isostructural chiral metal-organic frameworks decorated with chiral dihydroxy or -methoxy auxiliares from enantiopure tetracarboxylate-bridging ligands of 1,1′-biphenol and a manganese carboxylate chain. The framework bearing dihydroxy groups functions as a solid-state host capable of adsorbing and separating mixtures of a range of chiral aromatic and aliphatic amines, with high enantioselectivity. The host material can be readily recycled and reused without any apparent loss of performance. The utility of the present adsorption separation is demonstrated in the large-scale resolution of racemic 1-phenylethylamine. Control experiments and molecular simulations suggest that the chiral recognition and separation are attributed to the different orientations and specific binding energies of the enantiomers in the microenvironment of the framework. Chirality is one of the essential attributes of nature [1] . A wide variety of substances have their own stereoisomers, such as pharmaceuticals, nutraceuticals and agricultural chemicals, and the enantiomers often exhibit different biological and pharmacological responses [1] , [2] . Enantiomers remain a challenge to be separated owing to their identical physical and chemical properties in an achiral environment [3] . For decades, extensive research has been devoted to the development of chiral separation processes [3] , [4] . Resolution methods, with an emphasis on chromatographic separation and preferential crystallization, have been reported. While chromatography based on chiral stationary phases (CSPs) is a robust technology, it is expensive. The synthesis of CSPs with higher surface areas and multiple active sites are highly desired for high-performance resolutions [5] . Crystallization resolution outperforms other methods because of its low cost, high capacity and easy scale-up, but versatile chiral selectors are scarce [6] . Therefore, there is a critical need to develop a new generation of chiral materials with superior enantioseparation performance. The incorporation of enantiomerically pure building blocks into porous materials has been an ambitious goal and creates potential opportunities for enantioselective processes [7] . Although zeolites contain channels and cages of molecular dimensions and therefore are ideally suited for molecular separation, the preparation of enantiopure zeolites is very challenging [8] , [9] . As a new class of crystalline hybrid materials composed of organic linkers and metal ions, metal-organic frameworks (MOFs) have emerged as an ideal platform for engineering functional porous materials [10] , [11] , [12] , [13] , [14] , [15] . In particular, chiral MOFs are highly promising for the separation of enantiomers and for chiral catalysis, as a result of their high porosity, functional diversity, flexibility and size and shape selectivity, surpassing traditional inorganic and organic porous materials [16] , [17] , [18] , [19] , [20] . Chiral MOF catalysts with uniform active sites for enantioselective reactions have been developed based on functionalized chiral molecular (pre)catalysts [21] , [22] , [23] , [24] , [25] , [26] , [27] , [28] , [29] , [30] . In a handful of latest studies, the resolution of enantiomers (racemic alcohols and sulphoxides) with chiral MOFs via chromatography [31] , [32] , [33] , [34] , crystallization [35] , [36] , [37] , [38] , [39] , [40] and membrane [41] , [42] has been reported, but only few exhibit good chiral separation performance. Enantioseparations with porous materials are attractive but provide fundamental challenges in materials design. An important challenge associated with chiral MOFs as enantioselective adsorbents is how to create the driving force efficiently to discriminate two opposite enantiomers in an inclusion process [43] , [44] . Chiral recognition generally relies on a minimum of three simultaneous interactions between the selector and analyte—the so-called three-point rule [3] , [44] . At least one of these interactions must be stereoselective to form diastereomeric complexes and enable chiral separation. Therefore, the ability to achieve chiral recognition is pivotally important in controlling key events in enantioseparation. For a MOF to act an enantioselective selector, it should possess multiple chiral recognition sites that can work synergistically to induce selective recognition and binding of analytes and to exert stereocontrol. However, it is challenging to create the selectivity essential for separation of stereoselectively different forms of compounds [43] , [44] . We have demonstrated the separation of racemic alcohols by adsorption with MOFs and related assemblies [39] , [45] , [46] , [47] . Enantiomerically pure amines are key intermediates in a number of pharmaceutical compounds that possess a wide range of biological activities [48] . In comparison with alcohols, the resolution of amines is more challenging as amines are more reactive than alcohols and tend to dissociate MOF structures. To address this issue, C 2 -symmetric twisted tetracarboxylate ligands derived from 1,1′-biphenol were designed for the MOF synthesis. There are two hydroxyl groups in the ligand prearranged for enantioselectively recognitions after the MOF is formed, and two tert -butyl groups for facilitating stereochemical control. Here we report the synthesis of robust porous chiral MOFs constructed from H 4 L 1 (or H 4 L 2 ) and manganese carboxylate infinite chains ( Fig. 1 ), and their applications in enantioseparation of racemic primary and secondary amines by adsorption as well as liquid chromatography. Furthermore, molecular simulations are conducted to provide microscopic insights into experimentally observed enantioseparation. 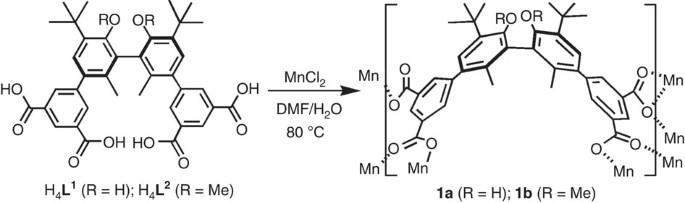Figure 1: Synthesis of the MOFs. Reaction of MnCl2·4H2O and H4L1or H4L2in a mixed solvent at elevated temperature afforded isostructural compounds1aand1b. Figure 1: Synthesis of the MOFs. Reaction of MnCl 2 ·4H 2 O and H 4 L 1 or H 4 L 2 in a mixed solvent at elevated temperature afforded isostructural compounds 1a and 1b . Full size image Synthesis and characterization of the MOFs The ligand H 4 L 1 was prepared by a Pd-catalysed Suzuki cross-coupling of dimethyl-5-(pinacolboryl)isophthalate and ( S )-3,3′-di- tert -butyl-5,5′-dibromo-6,6′-dimethylbiphenyl-2,2′-diol and followed by hydrolysis with LiOH. The ligand H 4 L 2 was obtained in 68% yield by protecting the ester of ( S )-H 4 L 1 with MeI and followed by base-catalysed hydrolysis. Pale yellow crystals of [Mn 2 L 1 (DMF) 2 (H 2 O) 2 ]·3DMF·2H 2 O ( 1a ) and [Mn 2 L 2 (DMF) 2 (H 2 O) 2 ]·3DMF·H 2 O ( 1b ) were obtained by heating MnCl 2 ·4H 2 O and H 4 L 1 or H 4 L 2 in DMF/H 2 O solution at 80 °C, respectively. The products were stable in air and insoluble in water and common organic solvents. The formulas of 1a and 1b were established by single-crystal X-ray diffraction (XRD), elemental analyses and thermogravimetric analysis (TGA). The uniformity of their bulk samples was established by powder XRD (PXRD). The values of molar optical rotation of the extracted ligands ( S )-H 4 L 1 and ( S )-H 4 L 2 from 1a and 1b digested by a dilute HCl solution are almost the same as the original values (~62° and −18°, respectively, c = 0.01 mol l −1 in dimethyl sulphoxide at 20 °C), suggesting the high stability of the chiral biphenyl configuration towards the crystallization conditions of MOF synthesis. ( S )- 1a crystallizes in the tetragonal chiral space group P 4 1 2 1 2. There are one L 1 ligand and two crystallographically independent Mn atoms in the asymmetric unit, with Mn1 and Mn3 sitting on the twofold screw axis (with one-half occupancies). Mn1 coordinates to two oxygen atoms of bridging carboxylate groups of L 1 ligands and two H 2 O and two DMF molecules, and Mn2 coordinates to five oxygen atoms of four bridging carboxylate groups and one DMF molecule, whereas Mn3 coordinates to four oxygen atoms of four bridging carboxylate groups and two H 2 O molecules in a distorted octahedral geometry. All of the three Mn centers adopt a distorted octahedral geometry and have normal Mn–O bond lengths (2.049(5)–2.319(4) Å). Mn1 and Mn2 are bridged by one bridging/bidentate carboxylate group, while Mn2 is linked to Mn3 by one bridging/bidentate and one bridging/chelate carboxylate groups ( Fig. 2 ). The Mn centers are thus linked by the bridging carboxylate groups to form one-dimensional chains having the formula [Mn 2 (CO 2 ) 2 ] n along the c axis, which act as the secondary building units for 1a . 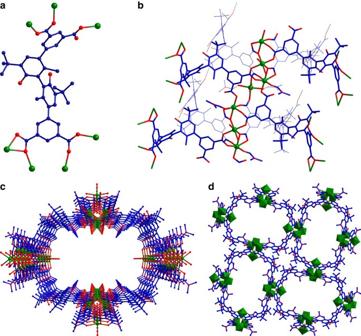Figure 2: X-ray structure of (S)-1a. (a) The coordination mode of theL1ligand. (b) The infinite Mn carboxylate chain. (c) Four metal-carboxylate chains linked by theL1ligands forming a 41helical channel. (d) View of the three-dimensional porous structure of (S)-1aalong thecaxis (the Mn atoms are shown in polyhedra). (Mn, green; O, red; N, purple; C, blue). Figure 2: X-ray structure of ( S )-1a. ( a ) The coordination mode of the L 1 ligand. ( b ) The infinite Mn carboxylate chain. ( c ) Four metal-carboxylate chains linked by the L 1 ligands forming a 4 1 helical channel. ( d ) View of the three-dimensional porous structure of ( S )- 1a along the c axis (the Mn atoms are shown in polyhedra). (Mn, green; O, red; N, purple; C, blue). Full size image The ligand L 1 exhibits an exo-heptadentate coordination fashion, in which the carboxylate groups show bridging/bidentate, bridging/chelate and monodentate modes ( Fig. 2a ), and its phenyl rings are twisted along the pivotal 1,1′-bond with a dihedral angle of 74(1)°. Four adjacent metal-carboxylate chains are bridged by biphenyl backbones of L 1 groups, which run around a 4 1 axis with a pitch of 13.0665(3)A˚, to give a nanosized tubule with an opening size of ~1.5 nm × 1.0 nm along the c axis (measured from van der Waals surfaces) ( Supplementary Fig. 1 ). Sharing of metal-carboxylate chains with neighbouring nanotubules leads to a chiral porous three-dimensional framework ( Fig. 2d ). The two dihydroxy groups of the ligand are partly shielded from the open channels by the biphenyl rings, but are still accessible to guest molecules. PLATON analysis revealed that the three-dimensional structure is composed of large solvent-accessible voids of 6729.9 Å 3 that constitute 46.1% volume per unit cell [15] . The crystal quality of complex 1b was too poor for a single-crystal structural determination to be performed, but cell parameter determination, PXRD and microanalysis studies established that 1b is isostructural to 1a ( Supplementary Fig. 2a ). Circular dichroism spectra of 1 made from R and S enantiomers of the H 4 L ligand are mirror images of each other, indicative of their enantiomeric nature ( Supplementary Fig. 3 ). TGA revealed that the guest molecules could be readily removed in the temperature ~100 °C, and the decomposition of the framework starts at ~400 °C ( Supplementary Fig. 4 ). Removal of guest molecules in the frameworks was achieved by replacing (via soaking) the initially present guest molecules with more volatile MeOH molecules followed by heating under vacuum. The crystallinity of the evacuated frameworks remains intact. The permanent porosity of 1a and 1b was confirmed by N 2 sorption isotherms at 77 K, as shown in Fig. 3 . Both of them exhibit type-I sorption behaviour, with Brunauer-Emmett-Teller (BET) surface areas of 2,145.0 and 1,746.0 m 2 g −1 , respectively ( Supplementary Fig. 5 ). Moreover, no significant loss of crystallinity was observed for 1a after soaking in water, methanol and toluene for one week, respectively ( Supplementary Fig. 2b ). The sample of 1a after treating by these solvents has a BET surface area of 1,885.2, 2,041.6 and 1,945.6 m 2 g −1 , respectively, further confirming its framework stability and permanent porosity ( Supplementary Fig. 6 ). The excellent chemical and thermal stability is consistent with their high connectivity networks bearing robust metal-carboxylate infinite chains as secondary building blocks. 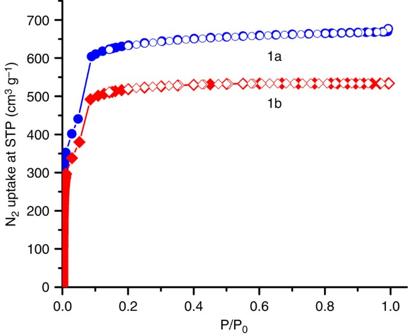Figure 3: N2sorption isotherms. N2adsorption isotherms (filled symbols) and desorption isotherms (open symbols) of MOF1a(blue) and1b(red) at 77 K. Figure 3: N 2 sorption isotherms. N 2 adsorption isotherms (filled symbols) and desorption isotherms (open symbols) of MOF 1a (blue) and 1b (red) at 77 K. Full size image Enantioselective adsorption and separation The presence of large chiral pores and available chiral dihydroxyl groups of biphenol in 1a prompted the exploration of enantioselective adsorption and separation. Initial studies identified the apohost 1a as an excellent adsorbent for amines, and a variety of resolution conditions was screened for selectivity with 1-phenylethylamine (1-PEA) as a model substrate. Upon solvent screening, the evacuated crystals of ( S )- 1a were immersed in racemic 1-PEA, in different solvents at room temperature for 2 h, filtered and washed with MeOH. Chiral high-performance liquid chromatography (HPLC) analysis of the desorbed 1-PEA showed that MeOH was the most suitable solvent for separation ( Table 1 , entries 1–6), allowing for 88.5% ee with the R -enantiomer being in excess, which was confirmed by comparing the retention time with that of the standard sample. Decreasing the temperature from 23 °C to 0 °C and to −10 °C led to better enantioselectivity, but further decreasing did not affect enantioselectivity and required a longer adsorption time ( Table 1 , entries 7–9). The chiral nature of the included molecule is determined by the handedness of the host, as further evidenced by the remarkable inclusion preference of ( R )- 1a for the S -enantiomer of 1-PEA over the R -enantiomer (88.3 % ee , Table 1 , entry 10) (HPLC spectrum see Supplementary Fig. 7 ). Kinetic study indicated that the adsorption of 1a to 1-PEA in MeOH reached equilibrium in 2 h ( Supplementary Fig. 8 ). Table 1 Enantiosorption of 1a to racemic 1-phenylethylamine. * Full size table With the optimized separation conditions established, we next examined the scope of the developed methodology with a variety of aromatic amines with different electronic and steric properties ( Fig. 4 ). First, a variety of electron-deficient and electron-rich substituents on the aromatic ring were investigated. Substitution in the para position of the aromatic ring ( 2b – 2d ) gave rise to the excellent enantioselectivity, regardless of the electronic nature of the substituent. Specially, 1-(4-fluorophenyl)ethylamine gave the highest ee value up to 98.3 % ( 2b′ ). In contrast, the o - and m -substituted 1-PEA ( 2e and 2f ) only gave moderate ee values. When the methyl group of 1-PEA was substituted with the ethyl group, the substrate 1-phenylpropylamine ( 2g ) was resolved with comparable enantioselectivity (92.3% ee ) to the parent amine, whereas the derivative indan-1-ylamine ( 2h ) exhibited a decrease in enantioselectivity (77.9% ee ). Thirdly, the hindered aromatic amine, 1-naphthalen-1-yl-ethylamine, was also tested for the resolution and 71.5% ee of 2i′ was obtained. Finally, 1-methyl-1,2,3,4-tetrahydroisoquinoline ( 2j ) and 1-methyl-3-phenylpiperazine ( 2k ), both of which are components of a number of chiral pharmaceuticals, were resolved with good levels of enantioselectivity up to 53.3 and 87.7% ee. HPLC spectra are supplied for 2a′-2k′ , see Supplementary Figs 9–19 . As a further demonstration of the utility of our adsorption separation, a large-scale resolution of 1-PEA was performed, yielding 116 mg of the product with 92.5% ee (HPLC spectrum see Supplementary Fig. 20 ). 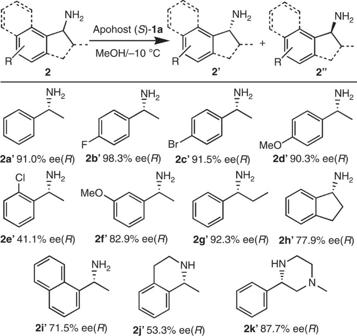Figure 4: Enantiosorption of (S)-1a towards benzyl amine and its derivatives. For details see Methods. Theeevalues were determined by HPLC (letters in brackets specify the preferable isomer). Figure 4: Enantiosorption of ( S )-1a towards benzyl amine and its derivatives. For details see Methods. The ee values were determined by HPLC (letters in brackets specify the preferable isomer). Full size image The excellent levels of asymmetric adsorption with aryl-substituted substrates encouraged us to examine alkyl amines and related derivatives, which are more difficult to separate than benzyl amines. Encouragingly, these substrates underwent the adsorption resolution with impressed enantioselectivities ( Fig. 5 ). For typical alkyl amines such as 2-butylamine 3a , 3-methyl-2-butylamine 3b , 2-pentylamine 3c and 1-cyclohexylethanamine 3d , they were strongly adsorbed by the apohost 1a and recovered quantitatively with enantioselectivity ranging from 76.1 to 85.1% ee . We have also evaluated two alkylamine derivatives. 1-Phenylpropan-2-amine 3e , a psychostimulant and sympathomimetic drug was resolved with 84.5% ee , whereas phenylalanine methyl ester 3f , an amino-acid derivative with an unprotected amino group, was resolved with enantioselectivity of 60.9% ee . HPLC spectra are supplied for 3a′-3f′ , see Supplementary Figs 21–26 . It is worth noting that in all cases the resolutions were conducted under identical conditions and only minor variations in the desorption workup were made. 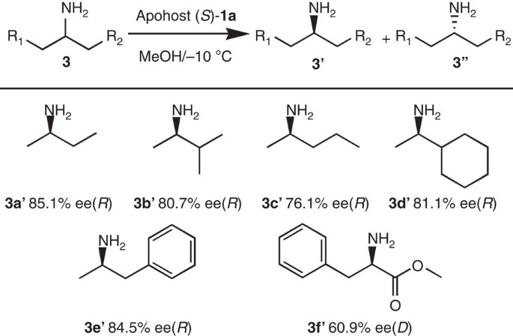Figure 5: Enantiosorption of (S)-1a towards aliphatic amines and related amines. For details see Methods. Theeevalues were determined by HPLC (letters in brackets specify the preferable isomer). Figure 5: Enantiosorption of ( S )-1a towards aliphatic amines and related amines. For details see Methods. The ee values were determined by HPLC (letters in brackets specify the preferable isomer). Full size image Typically, it took 1–2 h to reach diffusion equilibrium in enantioselective sorption even for bulkier substrates ( Supplementary Methods ). As expected, the bulkier 1-PEA has slower adsorption kinetics than the smaller 2-butylamine (1 and 2 h for the former and the latter, respectively). Elemental analysis and 1 H nuclear magnetic resonance (NMR) spectroscopy suggested the formation of target host–guest complexes, which can be formulated as [ 1a ·amine·MeOH·H 2 O] for 2-butylamine ( 3a ), 3-methyl-2-butylamine ( 3b ), 2-pentylamine ( 3c ), 1-cyclohexylethanamine ( 3d ) and as [ 1a ·amine·MeOH] for the other amines ( Supplementary Methods ). The smaller size of amines leads to a composition of one water guest molecule per formula unit of the host. It is likely that the sorption of amine guest correlates to the pair of available hydroxyl groups of biphenol per unit cell. To evaluate the stability of the solid adsorbent, we investigated recycled and reused 1a in the resolution of 1-(4-fluorophenyl)ethylamine. The adsorbent 1a could be recovered and used repeatedly without the deterioration of enantioselectivity for the following three runs (98.3, 98.7, 97.1 and 97.5% ee for runs 1−4, respectively). HPLC was performed: see Supplementary Figs 27–29 . The recycled sample of 1a remained highly crystalline and showed permanent porosity, with a BET surface area of 1927.7 m 2 g −1 ( Supplementary Figs 2c and 5c ). Inductively coupled plasma optical emission spectrometer (ICP-OES) analysis of the resolution solution indicated almost no loss of the Mn ion (<0.01%) from the structure in each cycle. HPLC separation MOF 1a- packed column for HPLC was prepared by loading the suspension of ( S )- 1a with an average size of ~5 μm in MeOH into a 25-cm-long × 2.0 mm internal diameter (i.d.) stainless steel column ( Supplementary Fig. 30 ). The performance of the CSP was first evaluated by enantioseparation of 1-PEA, but we failed to separate it. HPLC of the free amine is usually unsatisfactory owing to the strong adsorption of solutes on the column. Therefore, acylation of amines may be employed not only to reduce the polarity but also to improve the selectivity, sensitivity and separation of these amines. After optimizing mobile phase composition and its flow rate, racemic 1-PEA after benzoylation was successfully resolved and baseline separated on the CSP with hexane/isopropanol (optimized v/v=97:3) as the mobile phase at a flow rate of 1 ml min −1 at 23 °C ( Fig. 6a ). The high-resolution enantioseparation with a good selectivity factor ( α =1.4) and chromatographic resolution ( R s=2.7) was achieved within 30 min, and the elution sequence was the S -enantiomer followed by the R -enantiomer. 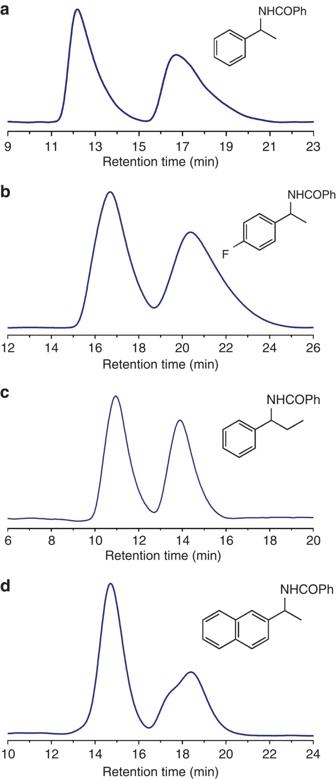Figure 6: HPLC separation of racemic amines on the 1a-packed column. (a) 1-phenylethylamine (b) 1-(4-fluorophenyl)ethylamine (c) 1-phenylpropylamine (d) 1-naphthalen-1-yl-ethylamine after benzoylation using hexane/isopropanol of ~90/10 (v/v) as the mobile phase at 23 °C, monitored with a ultraviolet detector at 254 nm. Figure 6: HPLC separation of racemic amines on the 1a-packed column. ( a ) 1-phenylethylamine ( b ) 1-(4-fluorophenyl)ethylamine ( c ) 1-phenylpropylamine ( d ) 1-naphthalen-1-yl-ethylamine after benzoylation using hexane/isopropanol of ~90/10 (v/v) as the mobile phase at 23 °C, monitored with a ultraviolet detector at 254 nm. Full size image Racemic 1-(4-fluorophenyl)ethylamine, 1-phenylpropylamine and 1-naphthalen-1-yl-ethylamine after benzoylation could also be baseline separated on the CSP with hexane/isopropanol (optimized v/v=98:2, 98:2 and 99:1, respectively) as the mobile phase, with a selectivity factor α =1.2, 1.3 and 1.2 and resolution R s=1.7, 2.2 and 2.1, respectively ( Fig. 6b–d ). Again, the elution sequence of each racemate was followed in the same order, the S -enantiomer always before the R -enantiomer. This order is consistent with the channels of ( S )- 1a prefer to include the R -enantiomer of amine over the S -enantiomer. After HPLC measurement, the sample PXRD pattern was obtained in accord with the as-synthesized solids before HPLC measurement ( Supplementary Fig. 2c ). The result proved that the crystals of 1a did not change its crystal structure when used as CSP for enantioseparation in HPLC. To examine the tolerating capability of the CSP without compromising resolution, a loading test was carried out using different injection mass. Even when the loading was increased from 4.0 to 20 μg, each racemate, for example, 1-PEA could still achieve baseline resolution ( Supplementary Fig. 31 ). This character of the CSP makes it possible to apply in preparative chromatogram. In addition, the chromatographic peak area of each single antipode rose linearly with the increase in the injected mass ( Supplementary Fig. 32 ). It was also evident that the retention time of the enantiomer for 1-PEA became closer with increasing injection mass from 4.0 to 20 μg, although achieving baseline resolution. Many artificial porous organic and hybrid hosts have been developed for chiral recognition and resolution of organic molecules, such as alcohols in a solid state, but there are few examples of enantioselective inclusion of amines [8] , [43] , [44] . In 1995, Mallouk et al . [49] pioneered optical resolution of amine (1,2-diaminocyclohexane, 85% ee) through intercalation by a layered phosphate with an optically active building block. In 2001, Lin et al . [50] reported resolution of racemic 1,2-diaminocyclohexane (13.6% and 10% ee for ( S,S )- and ( R,R )-1,2-diaminocyclohexane, respectively) on a flash chromatography using chiral laminar lanthanide phosphonates of BINOL as solid phases. For small secondary amines, such as 2-butylamine, it is difficult to recognize chirality because the subtle structural difference between the enantiomers as methyl groups and hydrogen atoms attached to the chiral carbon atom have to be discriminated. The present MOF represents a new generation of chiral porous solid that is capable of chiral separation of a variety of racemic amines. The success may result from a combination of the chiral channels with amphiphilic channel interior lined with chiral –OH auxiliaries, which may govern the intermolecular interactions between the host and amines favouring enantioselectivity during the adsorption process [43] , [44] , [51] . Unfortunately, attempts to get the single crystal of the inclusion adduct were unsuccessful. To evaluate the contribution of –OH groups of biphenol units in MOF 1a to the above chiral separation process, we examined the separation ability of MOF 1b that contains methyl-protected biphenol groups towards amines under otherwise identical conditions. In contrast to MOF 1a , the apohost 1b could adsorb both 2-butylamine and 1-PEA, but with essentially no enantioselectivity. Moreover, we also failed to separate 1-PEA and 1-phenylpropylamine using a HPLC column packed with 1b . Meanwhile, it is noted that the ligand methyl ester Me 4 L could also form a 1:1 adduct with 2-butylamine or 1-PEA by crystallization, but almost no enantioselectivity was observed for the examined amines. Overall, these results indicate that the chiral –OH groups of biphenol, together with the Mn atoms and phenyl rings create a microenvironment in the MOF, which is crucial for the optical discrimination of small organic molecules. Molecular simulations To provide microscopic insight into the origin of enantioselectivity of the amine adsorption, molecular simulations were conducted ( Supplementary Figs 33 and 34 ). 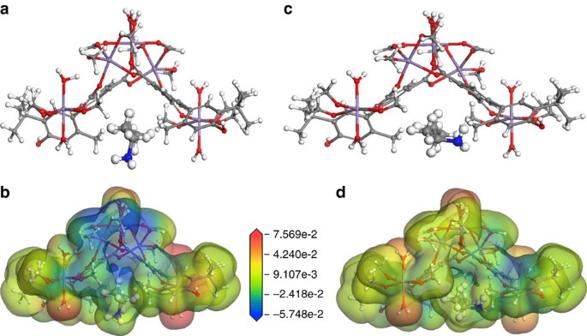Figure 7: Binding sites and electrostatic potential maps. (a,b) (R)-2-butylamine in (S)-1a(c,d) (S)-2-butylamine in (S)-1a. Figure 7 illustrates the binding sites and electrostatic potential maps for ( R )- and ( S )-2-butylamine enantiomers in MOF ( S )- 1a . Both enantiomers are preferentially located in the microenvironment formed by the –OH groups, Mn atoms and phenyl rings. However, the orientation and potential map of the ( R )-enantiomer are distinctly different from those of ( S )-enantiomer. Consequently, the specific binding energies are different, equal to −18.94 and −17.74 kcal mol −1 for ( R )- and ( S )-enantiomers, respectively. This indicates that ( R )-2-butylamine has a stronger interaction with ( S )- 1a than ( S )-counterpart. Figure 7: Binding sites and electrostatic potential maps. ( a , b ) ( R )-2-butylamine in ( S )- 1a ( c , d ) ( S )-2-butylamine in ( S )- 1a . Full size image The differences in orientation and binding energy are expected to cause enantioselective adsorption. Shown in Fig. 8 are the adsorption isotherms of racemic mixtures of ( R )-/( S )-2-butylamine in ( S )- 1a . Because of a stronger binding energy, ( R )-enantiomer is more predominantly adsorbed than ( S )-enantiomer, which is consistent with experiment. Our previous simulation studies [52] , [53] also revealed that the interaction between enantiomer and chiral adsorbent is crucial in enantioselective adsorption. Furthermore, Supplementary Fig. 35 illustrates the binging sites and electrostatic potential maps for 1-PEA enantiomers. Similarly, ( R )-1-PEA exhibits a different orientation and potential map from ( S )-1-PEA in the microenvironment, and the former possesses a stronger binding energy. As a consequence, ( R )-1-PEA is more preferentially adsorbed as shown in Supplementary Fig. 36 , which again is consistent with experiment. It is worthy to note that 1-PEA is bulkier in size compared with 2-butylamine, thus its adsorption capacity is lower. 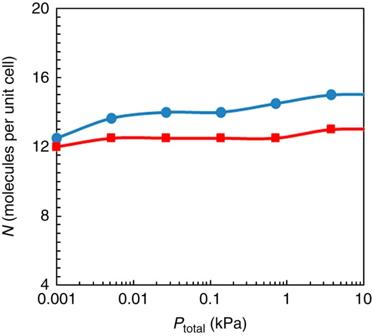Figure 8: Adsorption isotherms in (S)-1a. Enantioselective adsorption isotherms of racemic mixtures of (R)-/(S)-2-butylamine (blue circles/red squares). Figure 8: Adsorption isotherms in ( S )-1a. Enantioselective adsorption isotherms of racemic mixtures of ( R )-/( S )-2-butylamine (blue circles/red squares). Full size image We have presented two homochiral robust 1,1′-biphenol-based MOFs that contain one-dimensional nanosized channels decorated with chiral dihydroxyl or dimethoxy groups. The materials exhibit high thermal stability and framework robustness as well as permanent porosity. The framework containing chiral dihydroxyl auxiliaries can be utilized as adsorbents for the separation of racemic aromatic and aliphatic amines, and as a CSP of HPLC for the enantioseparation of racemic amines. Experimental and simulation results revealed that the intrinsic chiral recognition and separation are attributed to the different orientations and binding energies of the two enantiomers within the microenvironment of the MOF. Such highly enantioselective separation, synergizing the latest development in nanoporous materials and achievement in adsorption technology, has not been reported to date. This work may bring advanced materials science and engineering to the forefront of practical application and a major societal need. Materials and general procedures All reagents and solvents used in these studies are commercially available and used without further purification. 1 H and 13 C NMR experiments were carried out on a MERCURYplus 400 spectrometer operating at resonance frequencies of 400 MHz. 1 H NMR and 13 C NMR spectra are supplied for ( S )-H 4 L 1 , ( S )-H 4 L 2 and corresponding intermediates: see Supplementary Figs 37–40 . Elemental analyses of C, H and N were performed with an EA1110 CHNS-0 CE elemental analyzer. The infrared (IR) (KBr pellet) spectra were recorded (400–4,000 cm −1 region) on a Nicolet Magna 750 fourier transform IR spectrometer. The solid-state circular dichroism spectra were recorded on a J-800 spectropolarimeter (Jasco, Japan). TGA were carried out in an air atmosphere with a heating rate of 10 °C min −1 on a STA449C integration thermal analyzer. PXRD data were collected on a DMAX2500 diffractometer using Cu Kα radiation. The calculated PXRD patterns were produced using the SHELXTL-XPOW program and single-crystal reflection data. ICP-OES was performed on Optima 7300DV ICP-OES (Perkin Elmer Coporation, USA). Electrospray ionization mass spectra were recorded on a Finnigan LCQ mass spectrometer using dichloromethane-methanol as mobile phase. Electrospray ionization mass spectra are supplied for ( S )-H 4 L 1 and ( S )-H 4 L 2 : see Supplementary Fig. 41 . Analytical HPLC was performed on a YL-9100 HPLC with ultraviolet detection at 220 nm. Analytical CHIRALCEL OD-H columns (4.6 mm × 25 cm) from Daicel were used. See Supplementary Methods for the procedures and characterization data of compounds not listed in this part. X-ray crystallography Single-crystal XRD data for the compound was collected on a Bruker Smart APEX II CCD diffractometer with Cu-Kα radiation ( λ =1.54178 Å) at 123 K. The empirical absorption correction was applied by using the SADABS program (G.M. Sheldrick, SADABS, program for empirical absorption correction of area detector data; University of Göttingen, Göttingen, Germany, 1996). The structure was solved using a direct method, and refined by full-matrix least-squares on F2 (G.M. Sheldrick, SHELXTL97, program for crystal structure refinement, University of Göttingen, Germany, 1997). A full set of data was collected; however, the very high-angle data was dominated by noise and was omitted, resulting in the value of sine (theta_max)/wavelength of 0.4968. Owing to the weak diffraction, hydrogen atoms of water could not be located from difference Fourier map and all of the phenyl rings are constrained to ideal six-membered rings. All non-hydrogen atoms are refined anisotropically, except for the guest molecule water. Elemental analysis showed that the formula unit of 1a includes three DMF and two water guest molecules. See Supplementary Data 1 ; Supplementary Tables 1–2 . Synthesis of ( S )-1a and ( S )-1b A mixture of MnCl 2 ·4H 2 O (12 mg, 0.06 mmol), the ligand ( S )-H 4 L 1 or ( S )-H 4 L 2 (0.03 mmol), MeOH (5 ml), DMF (1 ml) was sealed in a 10-ml vial with a screw cap and heated at 80 °C for 1 day. Pale yellow crystals of ( S )- 1a and ( S )- 1b were collected, washed with ether and dried in air (78% yield for ( S )- 1a and 75% for ( S )- 1b , based on the ligand). Elemental analysis (%): calcd for [Mn 2 L 1 (DMF) 2 (H 2 O) 2 ]·3DMF·2H 2 O ( 1a , C53H77Mn2N5O19): C, 53.13; H, 6.48; N, 5.85. Found: C, 52.79; H, 6.34; N, 5.74; fourier transform IR (KBr pellet, cm −1 ): 3.513(m), 3,389(m), 2,959(m), 2,850(w), 1,613(m), 1,554(s), 1,444(m), 1,410(m), 1,365(s), 1,258(w), 1,172(m), 1,128(w), 1,034(w), 923(w), 897(w), 784(w), 719(w), 679(w), 637(w), 592(w), 479(w). Elemental analysis (%): calcd for [Mn 2 L 2 (DMF) 2 (H 2 O) 2 ]·3DMF·H 2 O ( 1b , C55H79Mn2N5O18): C, 54.68; H, 6.59; N, 5.80;. Found: C, 54.00; H, 6.52; N, 5.74. FTIR (KBr pellet): 3,394(m), 2,957(m), 2,870(w), 1,659(m), 1,618(m), 1,553(s), 1,439(m), 1,417(m), 1,367(s), 1,303(w), 1,249(w), 1,223(w), 1,108(w), 1,059(w), 970(w), 925(w), 871(w), 783(w), 724(w), 682(w), 624(w), 576(w). Unit cell parameter for ( S )- 1b : a=b=33.4210(10) Å, c=13.1020(10) Å, α = β = γ =90 o , V =14634.5(13) Å 3 . The guest molecules can be readily exchanged with ether and then evacuated at 100 °C for 4 h to generate the apohost ( S )- 1a and ( S )- 1b , as confirmed by TGA. General procedure for amine adsorption and separation Evacuated sample of ( S ) -1a (30 mg) and racemic amine (0.01 ml) in MeOH (5 ml) were mixed together in a sealed vial at −10 °C for ~2 h. The solid sample was filtered, washed with MeOH and then washed several times with THF or ether to give the encapsulated amines. The completeness of the substrate extraction was confirmed by 1 H NMR (Supplementary Fig. 42) and the N 2 sorption isotherm ( Supplementary Fig. 5 ). Optical purity of the desorbed amines was analysed via benzoylation (or acetylation) as described below, then determined by HPLC with a Chiralcel OD-H column (4.6 mm × 25 cm). To a solution of the encapsulated amine in THF (5 ml) was added Et 3 N (2 drops) and BzCl (or AcCl) (1 drops) at room temperature. The resulting reaction mixture was stirred for 2 h then diluted with Et 2 O (10 ml), washed with aqueous HCl (1M, 2 ml) and saturated NaCl solution, dried over anhydrous Na 2 SO 4 and concentrated in vacuum. The amine-exchanged solid of ( S) - 1a ·guest was carefully dried and the adduct composition was established by combination of 1 H NMR and elemental analysis. We failed to determine the adduct composition using TGA, probably owing to strong host–guest interactions. A large-scale experiment that afforded 116 mg of 1-PEA (92.5% ee in R excess) was conducted in a similar procedure using 1,000 mg ( S )- 1a for adsorption of racemic 1-PEA. Column packing procedure for HPLC measurement The CSP of 1a for HPLC was prepared by the upward stirred slurry method. The solvent-exchanged 1a was crushed in ethanol applying soft pressure and suspended in a mixture of hexane and dichloromethane. The suspension was packed into a 25-cm-long × 2.0 mm i.d. stainless steel column under 40~50 MPa. By varying the pressure to press the slurry into the column, the crystals could dispose slowly to get a better packing, and then the MOF column was obtained. The column was rinsed and equilibrated with the mobile phase before use. HPLC experiments were performed at 23 °C with a Shimadzu HPLC system (Shimadzu Corporation, Kyoto, Japan). It consists of a 20-A pumps and a variable-wavelength ultraviolet detector. Data acquisition and processing were performed on a N2000 chromatography data system. The injection volume and the flow rate were 5 μl and 1 ml min −1 , respectively. The wavelength of ultraviolet detection was 254 nm. Separation factor ( α ) and resolution factor ( Rs ) were obtained from the following equations: where t R 1 and t R 2 represent the retention times of right- and left-handed enantiomers ( t R 2 > t R 1 ), W 1 and W 2 are the widths of the bases formed by triangulation of the peaks, respectively. Molecular simulations The models for the MOF 1a and two amines (2-butylamine and 1-PEA) are described in the Supplementary Information . To identify the preferential binding site for each enantiomer, simulation annealing was conducted in a canonical ensemble with temperature decreased from 1,000 to 100 K. The simulation box contained two (1 × 1 × 2) unit cells of the MOF and a single amine molecule. The MOF was assumed to be rigid and the framework atoms were fixed during simulation. The Lennard–Jones interactions were evaluated by the atom-based method with a spherical cutoff of 13 Å and a cubic spline width of 1.0 Å, while the Coulombic interactions were calculated using the Ewald summation method with an accuracy of 10 −4 kcal mol −1 . To estimate the adsorption of equimolar racemic mixtures, grand canonical Monte Carlo (GCMC) simulation was conducted at 263 K. The number of steps in the GCMC simulation was 10 6 , and followed by 10 5 production steps. Five types of trial moves were randomly attempted in the GCMC simulation: exchange, conformer, translation, rotation and regrowth. Accession codes: The X-ray crystallographic coordinates for the structures reported in this article have been deposited at the Cambridge Crystallographic Data Centre (CCDC), under deposition number CCDC 869399. These data can be obtained free of charge from The Cambridge Crystallographic Data Centre via http://www.ccdc.cam.ac.uk/data_request/cif . How to cite this article: Peng, Y. et al . Engineering chiral porous metal-organic frameworks for enantioselective adsorption and separation. Nat. Commun. 5:4406 doi: 10.1038/ncomms5406 (2014).